High-strength and thermally stable bulk nanolayered composites due to twin-induced interfaces Bulk nanostructured metals can attribute both exceptional strength and poor thermal stability to high interfacial content, making it a challenge to utilize them in high-temperature environments. Here we report that a bulk two-phase bimetal nanocomposite synthesised via severe plastic deformation uniquely possesses simultaneous high-strength and high thermal stability. For a bimetal spacing of 10 nm, this composite achieves an order of magnitude increase in hardness of 4.13 GPa over its constituents and maintains it (4.07 GPa), even after annealing at 500 °C for 1 h. It owes this extraordinary property to an atomically well-ordered bimaterial interface that results from twin-induced crystal reorientation, persists after extreme strains and prevails over the entire bulk. This discovery proves that interfaces can be designed within bulk nanostructured composites to radically outperform previously prepared bulk nanocrystalline materials, with respect to both mechanical and thermal stability. Future energy and defence applications require high-strength and robust materials that can maintain their properties under extreme conditions of temperature, strain and strain rate. Promising material candidates for these applications are nanostructured materials. Pure single-phase nanocrystalline materials have outstanding mechanical properties [1] , [2] , [3] , [4] , [5] , but they are not thermally stable because they are inherently comprised of a high fraction of grain boundaries that are disordered in structure and high in boundary energy [6] , [7] . Alloying [8] has been proposed to surmount the thermal stability problem. However, less attention has been paid to nanostructured multi-phase materials, which contain a higher density of heterophase interfaces than grain boundaries [9] , [10] , [11] , [12] , [13] . Of particular interest are composites comprised of two phases that do not chemically mix, leading to bimetal interfaces that are sharp and potentially ordered in atomic structure [14] . The ability to achieve such structural order opens up an alternative route for materials design involving tuning the physical properties of the bimetal interfaces rather than those of the phase(s). Success, however, relies on knowing a priori which interface structures are mechanically and thermally desirable and how to control composite synthesis to achieve them. Fabrication of nanostructured bulk metals with high interface content has been achieved in many ways [15] , [16] , [17] , [18] , [19] , [20] , [21] , [22] , [23] , and in some cases particular interfaces have been created [20] , [21] , [22] , [23] . One important example of a successful application of grain boundary engineering [24] is the fabrication of nanotwinned copper, in which the high-strength microstructure contains nanotwins separated by finely spaced twin boundaries. Achieving peak strength relies upon stability of coherent twin boundaries and their ability to act as either effective barriers to dislocation motion or sources for dislocations [25] , [26] , [27] . The high stability of the coherent twin boundary also makes the nanotwinned structure thermally stable down to ~10 nm in twin width and up to 400 °C ( [22] ). However, formation of twin boundaries is only one of two ways twins affect material response. Twins also create a domain of material that has been significantly reoriented. In particular, when deformation twins exceed a critical volume fraction, they can greatly impact material texture, dislocation slip and deformation twin activity, and anisotropy in strength [21] , [28] , [29] , [30] , [31] . In this work, nanolamellar Cu/Nb composites in the form of bulk sheet with high interfacial content are fabricated via accumulative roll bonding (ARB) [32] (see Supplementary Fig. S1 ). ARB technology [33] is a severe plastic deformation (SPD) process that consists of repeated rolling, sectioning, stacking, bonding and re-rolling. We reveal that lattice reorientation due to twinning within the Cu/Nb bulk nanocomposites can be used to synthesize a remarkably mechanically and thermally stable bimetal interface. The twinning mechanisms are correlated to dislocation-twin transmission across the interface and/or interface dislocation dissociation. The composite with a bimetal spacing of 10 nm achieves a hardness of 4.13 GPa and maintains it (4.07 GPa), even after annealing at 500 °C for 1 h. The outstanding stability can be attributed to the energetically favourable nature of the atomically well-ordered bimetal interfaces. Texture evolution characterized by neutron diffraction Bulk neutron diffraction measurements of texture evolution from layer thickness h =200–10 nm indicate that Cu twinning unexpectedly occurs profusely throughout the material. 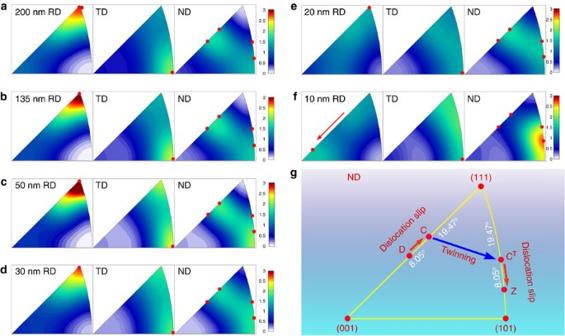Figure 1: Texture evolution due to twinning. (a–f) IPFs of the Cu layers within the ARB material with individual layer thicknesses of 200, 135, 50, 30, 20 and 10 nm, respectively; (g) a schematic of the reorientation pathway taken by the Cu crystals with strain, reducing the layer thickness from 200 to 10 nm. Texture components marked with red spots are C: {112} <111> and the twinning orientations CT: {552} <115>, D: {4 4 11} <11 11 8> and Z: {5 5 1} <1 1 10>. In particular, the spot in the RD-IPF offshows the new RD <1 1 10> at 10 nm layer thickness. Figure 1a–f presents the texture change in the Cu phase in the form of inverse pole figures (IPFs) for the rolling direction (RD), transverse direction (TD) and normal direction (ND), where the latter in particular is indicative of changes in the interface planes. Main texture components, Copper (C) {112}<111> and its {111} twinning orientation C T {552} <115>, Dillamore (D) {4 4 11} <11 11 8> and {5 5 1} <1 1 10> labelled by Z hereinafter, are marked with red symbols in the IPFs and Fig. 1g , which is a schematic of the ND-IPF. The corresponding texture in the Nb phase has a peak near {112}<110> that sharpens further with strain (see Supplementary Fig. S2 ). For h =200 and 135 nm, the Cu orientation distribution is predominantly oriented between D and C, being closer to D. At h =50 nm, the intensities of components C and C T have noticeably increased. From h =50–10 nm, when C T increases, the original C has depleted, and has been almost fully replaced by another highly oriented state at the Z {551}<1 1 10> orientation at h =10 nm. The texture evolution route resulting from twinning is illustrated in Fig. 1g . Figure 1: Texture evolution due to twinning. ( a – f ) IPFs of the Cu layers within the ARB material with individual layer thicknesses of 200, 135, 50, 30, 20 and 10 nm, respectively; ( g ) a schematic of the reorientation pathway taken by the Cu crystals with strain, reducing the layer thickness from 200 to 10 nm. Texture components marked with red spots are C: {112} <111> and the twinning orientations C T : {552} <115>, D: {4 4 11} <11 11 8> and Z: {5 5 1} <1 1 10>. In particular, the spot in the RD-IPF of f shows the new RD <1 1 10> at 10 nm layer thickness. Full size image Interface evolution characterized by transmission electron microscopy The texture evolution and unusual amounts of Cu twinning described above can be correlated to interface evolution via transmission electron microscopy (TEM) observation in the TD direction. As seen in Fig. 2a–f , the Cu/Nb interfaces in nanocomposites ( h <200 nm) after SPD are sharp and planar such that the ND of the sheet coincides with the planes of the Cu/Nb interfaces. Additionally, the alternating Cu/Nb lamellar structure has been demonstrated by high angle annular dark field scanning transmission electron microcopy (HAADF-STEM) (see Supplementary Fig. S3 ). For h <200 nm, the layers are single crystal through the thickness. Most remarkably, the material self organizes to a narrow set of predominant interfaces near {4 4 11}<11 11 8>Cu (D)||{112}<110>Nb, and including some fraction of {112}<111>Cu(C)||{112}<110>Nb interfaces. A rationale for its development was recently proposed [34] . When h refines to 50 nm, the amount of the {112}<111>Cu (C)||{112}<110>Nb interface increases and twins form in the Cu layers [35] , [36] . The two aforementioned interfaces are ordered, containing regular arrays of facets and interfacial dislocations to accommodate the lattice mismatch between the phases [36] , [37] , [38] (see Supplementary Fig. S4 ). These facets are an intrinsic structural feature and have been seen in interfaces with this same crystallography but different material systems [37] , [39] . From h =50 to 10 nm, the Cu twins increase in frequency, expand and coalesce (see Supplementary Fig. S5 ). As shown in Fig. 2f , at h =10 nm, most of the C component twinned and almost no twin boundaries are apparent. Consequently, the Cu crystal reorients from C to C T ( Fig. 1g ). When the Cu crystal twins while the Nb crystal remains fixed, the interface changes boundary character. 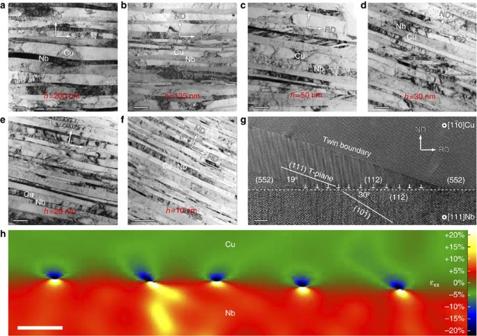Figure 2: Interface and twinning characterized by TEM. (a–f) TEM images showing that the lamellar structure of the ARB samples is maintained for the different layer thicknesses. Deformation twins become evident when the layer thickness reduces to about 50 nm. The twin volume fraction continues to increase as deformation proceeds further until the Cu layers are significantly reoriented at layer thickness of 10 nm. (g) A magnification of a twinning example in the sample with 30 nm layer thickness, showing the initial interface {112}<111>Cu||{112}<110>Nb and the interface {552}<115>Cu||{112}<110>Nb after twinning. (h) A GPA strain map of the (112)Cu||(11)Nb interface in (g) exhibiting misfit dislocation cores with sharp strain gradient. Scale bars: (a–b) 200 nm, (c–f) 100 nm, (g) 2 nm, (h) 1 nm. Figure 2: Interface and twinning characterized by TEM. ( a – f ) TEM images showing that the lamellar structure of the ARB samples is maintained for the different layer thicknesses. Deformation twins become evident when the layer thickness reduces to about 50 nm. The twin volume fraction continues to increase as deformation proceeds further until the Cu layers are significantly reoriented at layer thickness of 10 nm. ( g ) A magnification of a twinning example in the sample with 30 nm layer thickness, showing the initial interface {112}<111>Cu||{112}<110>Nb and the interface {552}<115>Cu||{112}<110>Nb after twinning. ( h ) A GPA strain map of the (112)Cu||(11 )Nb interface in ( g ) exhibiting misfit dislocation cores with sharp strain gradient. Scale bars: ( a – b ) 200 nm, ( c – f ) 100 nm, ( g ) 2 nm, ( h ) 1 nm. Full size image Twinning mechanism A high-resolution TEM (HRTEM) image in Fig. 2g shows an example of twinning from the {112}<111>fcc||{112}<110>bcc interface in a sample that has not yet fully twinned ( h =30 nm), and demonstrates how, within the twin domain, the interface has reoriented to {552}<115>fcc||{112}<110>bcc. The twinning plane (T-plane) in Cu is (111) tilted ~19.5° from the interface. This interface supports the nucleation of twins on the T-plane by two unit mechanisms: dislocation-twin transmission across the interface [35] , [36] , [40] and twin nucleation from the interface directly [36] , [41] . Both are only possible on the T-plane. Regarding the transmission mechanism, the T-plane is the only one that is well aligned across the interface with an active Nb {110} plane, as marked in Fig. 2g , meaning that the angle between the incoming and outgoing Burgers vector is minimal, and the Nb glide plane and T-plane share the common intersection line with the interface [36] . The other {111} T-planes in Cu, however, do not form such geometrically efficient dislocation transmission pathways with the active {110} or {112} planes in Nb and thus are not favoured. Regarding nucleation, the misfit dislocations with Burgers vectors of 1/3[111] Cu, marked on the (112)Cu||(11 )Nb interface in Fig. 2g , are able to dissociate into twinning partials on the T-plane [36] . Dissociation onto other twin planes is not possible as their intersection lines with the interface are not aligned with the line orientation of the misfit dislocations. To clearly display the interface dislocations in the (112)Cu||(11 )Nb interface in Fig. 2g , a strain map obtained by geometric phase analysis (GPA) [42] is provided in Fig. 2h . Once formed, fine twins first propagate across the Cu layer. They then expand laterally via a combination of the above two mechanisms [36] . The flat interface observed after twinning in Fig. 2g is evidence that twin expansion involved a combination of twinning partials with different Burgers vectors, such that when averaged over a sufficient length of the boundary, the net Burgers vector of twinning partials is zero [36] (see Supplementary Fig. S6 ). This method of expansion is expected to be more energetically favourable than continual sequential emission of the same Burgers vector from one side of the boundary, as it requires little to no accommodation by the adjoining Nb crystal. This mechanism shares the same principle as the formation of zero-strain twins [43] . Eventually twins expand within the layers and the new twin-induced Cu/Nb interface is created. Interface effects on texture and interface evolutions Thus far, we have reported that as layers refine from ultra-fine scales (>100 nm) to nanoscales (10 nm), the interface changes substantially from lying close to {4 4 11}<11 11 8>Cu (D)||{112}<110>Nb to {551}<1 1 10>Cu (Z)||{112}<110>Nb. We also observe that deformation twinning in the Cu has a key role in this interface change, namely that the {112}<111>Cu||{112}<110>Nb interfaces drive twinning and cause the interface to reorient to {552}<115>Cu||{112}<110>Nb. With the addition of atomistic simulation and crystal plasticity theory, the complete, multi-step reorientation pathway underlying the observed interface changes and the contribution that the twinning step makes can be clarified. As mentioned, at ultra-fine length scales, a persistent interface forms, wherein the Cu crystal orientation lies between D and C ( Fig. 1a ) and the adjoining Nb crystal near {112}<110>. The well-ordered atomic structure of this interface is shown in HRTEM images ( Fig. 3a ). Atomic scale simulation predicts that this predominant interface corresponds to local minima in interfacial energy (see Method: MD simulation Supplementary Table S1 and Supplementary Method : MD simulation), thus partly explaining its predominance at ultra-fine scales when bimetal interface density is high. However, as layer thickness reduces substantially to 50 nm and below, this interface, which was stable at submicron scales, becomes unstable. It can be expected that at such fine nano scales, the dislocation sources are limited within the phase, and dislocations are then supplied from the interface or by slip transmission across the interface. Once interface slip transmission controls slip dynamics within the crystals, the {4 4 11}<11 11 8>Cu (D)||{112}<110>Nb interface cannot be expected to maintain mechanical stability as it possesses only one effective slip transmission pathway between Cu and Nb (from the (10 ) Nb plane to the green (111) Cu plane in Fig. 3a ). Plastic slip in the Cu crystal consequently becomes asymmetric, occurring predominantly on the green (111) plane. This change in slip activity causes the interface to change from {4 4 11}<11118>Cu(D)||{112}<110>Nb to {112}<111>Cu(C)||{112}<110>Nb ( Fig. 1c ) [44] . Once the interface changes to {112}<111>Cu(C)||{112}<110>Nb, it easily twins on the same (111) T-plane, reorienting the interface to {552}<115>Cu||{112}<110>Nb ( Fig. 1e ). An HRTEM image of interface structure corresponding to {552}<115>Cu||{112}<110>Nb is shown in Fig. 3c . The {552}<115> orientation of Cu is unstable in rolling and, thus, further deformation drives the {552}<115>Cu||{112}<110>Nb interface to reorient via slip to {551}<1110>Cu (Z)||{112}<110>Nb ( Fig. 1f ; see Supplementary Fig. S7 ). By h =10 nm, the prevailing {551}<1110>Cu (Z)||{112}<110>Nb interface has been achieved. Note that during the multi-step path described above, Nb maintains the orientation {112}<110> as within it, plastic slip is symmetric. 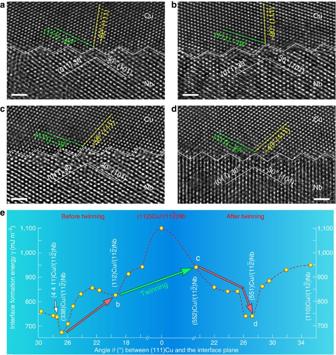Figure 3: Typical interface structures and their energies. (a–d) HRTEM images showing the typical interfaces with the beam direction along <110>Cu||<111>Nb, before twinning (a) (4 4 11)Cu||(11)Nb and (b) (112)Cu||(11)Nb, and after twinning (c) (552)Cu||(11)Nb and (d) (551)Cu||(11)Nb. The favoured fcc/bcc slip system pair for interface transmission is marked in green lines in Cu. (e) A profile of the excess energy of the interface as calculated by atomic-scale simulation with respect to the tilt angle about the <110>Cu from interface plane to the (111) plane in Cu. The orange lines represent reorientation predominantly by slip and the green line reorientation primarily by twinning. The calculation indicates that the final {551}<1 1 10>Cu ||{112}<110>Nb interface is energetically favourable, corresponding to a local minimum {338} is only 0.72° from D {4 4 11}, and both of them lie in the region of peak intensity in the IPFs for 200 nm (Fig. 1a) and 135 nm (Fig. 1b). Scale bars, 1 nm. Figure 3: Typical interface structures and their energies. ( a – d ) HRTEM images showing the typical interfaces with the beam direction along <110>Cu||<111>Nb, before twinning ( a ) (4 4 11)Cu||(11 )Nb and ( b ) (112)Cu||(11 )Nb, and after twinning ( c ) (552)Cu||(11 )Nb and ( d ) (551)Cu||(11 )Nb. The favoured fcc/bcc slip system pair for interface transmission is marked in green lines in Cu. ( e ) A profile of the excess energy of the interface as calculated by atomic-scale simulation with respect to the tilt angle about the <110>Cu from interface plane to the (111) plane in Cu. The orange lines represent reorientation predominantly by slip and the green line reorientation primarily by twinning. The calculation indicates that the final {551}<1 1 10>Cu ||{112}<110>Nb interface is energetically favourable, corresponding to a local minimum {338} is only 0.72° from D {4 4 11}, and both of them lie in the region of peak intensity in the IPFs for 200 nm ( Fig. 1a ) and 135 nm ( Fig. 1b ). Scale bars, 1 nm. Full size image Features of finial stable interface It is relevant to ask why the Z {551}<1 1 10>Cu ||{112}<110>Nb interface is the stable end point after extreme straining. HRTEM analysis of this interface in Fig. 3d reveals that it is intact, ordered and faceted, containing a regular array of interfacial dislocations (see Supplementary Fig. S8a ). This structure agrees with that calculated via atomistic simulations (see Supplementary Fig. S8b ). The consistency between the atomistic simulation for an undeformed interface and the actual interface in the heavily deformed sample indicates that the interface structure seen in the HRTEM is remarkably free of extrinsic defects despite having experienced over 1,000% strain. Atomistic simulations also find that the interface will be thermodynamically driven to {551}<1110>fcc ||{112}<110>bcc in order to lower the interface energy as shown in Fig. 3e . Furthermore, Fig. 3d shows that two symmetrically oriented Cu/Nb transmission pathways across this interface exist, which would ensure that adjoining Cu and Nb crystal orientations would remain stable with further rolling strain. These are consequences of interface-controlled mechanics because without considering the interface it would be expected that Cu crystal alone in either the {552}<115> or {551}<1110> orientation would immediately rotate to {110}<001>, which has a perfectly symmetric slip orientation [45] . High strength and thermal stability The interfaces not only impart outstanding mechanical stability, but also superior mechanical strength and thermal stability as revealed in Fig. 4 . Mechanical strength and thermal stability of the nanocomposites were examined by nanohardness testing and high temperature annealing. The hardness of the h =10 nm composites is 4.13±0.4 GPa, which is higher than that of gas-deposited nanocrystalline Cu with 15 nm grain size (2.4 GPa) [46] and that of physical vapour-deposited (PVD) nanotwinned Cu with 4 nm twin spacing (3.5 GPa) [22] , and approaches that of PVD Cu/Nb multilayers with layer thickness of 15 nm (5.3 GPa) [47] . After annealing at 500 °C for 1 h, the h =10 nm composites retain a hardness of 4.07±0.2 GPa. For the same size scale, they are as stable as PVD nanotwinned Cu ( [22] ) and PVD Cu/Nb multilayers [47] , and offer improved stability over gas-deposited nanocrystalline Cu [46] and PVD Mo/Pt multilayers [48] . As revealed in Fig. 4a , among all these composites, the present Cu/Nb nanocomposites have the smallest reduction in hardness. 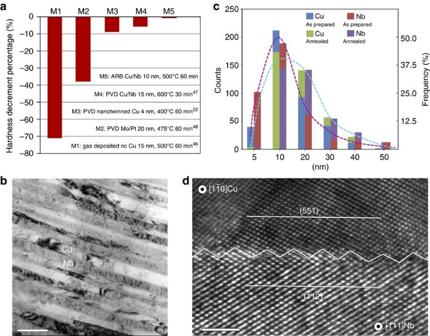Figure 4: Hardness and thermal stability at a layer thickness of 10 nm. (a) Decrease in hardness after annealing at elevated temperature from that at room temperature for several nanostructured materials found in the literature22,46,47,48. Notice that the present material, ARB Cu/Nb (10 nm), experiences the lowest drop in hardness and hence the best thermal stability; (b) a TEM image showing that the morphology after annealing at 500 °C for 1 h maintains the lamellar feature; (c) variation of layer thickness in the as prepared samples and the samples after the annealing, in which the columns representing the same elements overlap with the larger one placed behind. The dashed lines are the fitted distributions of layer thickness. Scale bars, 100 and 2 nm (forbandd, respectively). Figure 4: Hardness and thermal stability at a layer thickness of 10 nm. ( a ) Decrease in hardness after annealing at elevated temperature from that at room temperature for several nanostructured materials found in the literature [22] , [46] , [47] , [48] . Notice that the present material, ARB Cu/Nb (10 nm), experiences the lowest drop in hardness and hence the best thermal stability; ( b ) a TEM image showing that the morphology after annealing at 500 °C for 1 h maintains the lamellar feature; ( c ) variation of layer thickness in the as prepared samples and the samples after the annealing, in which the columns representing the same elements overlap with the larger one placed behind. The dashed lines are the fitted distributions of layer thickness. Scale bars, 100 and 2 nm (for b and d , respectively). Full size image Generally, the materials fabricated by deposition are expected to contain relatively low-energy interfaces as the deposition processes are in near thermal equilibrium, while materials synthesized by SPD are expected to contain high-energy, ‘thermally non-equilibrium’ interfaces [49] . Consistent with this viewpoint, nanocrystalline Cu prepared by high-pressure torsion (HPT), a SPD process, suffers grain coarsening and decreases in hardness even at 50 °C (ref. 18 ). In contrast, the ARB Cu/Nb composites, which are also fabricated via SPD, show great thermal stability, compared with that of materials prepared by deposition methods, while possessing superior strength. Figure 4b shows that the sample maintains its multilayer morphology, with flat and sharp interfaces, even after annealing with h =10 nm. Although, as shown in Fig. 4c , the layer thicknesses increase by a small amount and their distribution broadens slightly, the composites maintain the {551}<1110>Cu||{112}<111>Nb interface and its faceted features ( Fig. 4d ). In summary, we demonstrate that bulk two-phase nanocomposites fabricated via SPD contain an ultra-high density of a highly ordered bimetal interface {551}<1110>Cu||{112}<111>Nb, which is an outcome of atypically profuse deformation twinning. The crystallographic and energetic stability of this interface is found to enable ultrahigh strength and exceptional thermal stability of the nanocomposite. Such remarkable stability at mechanical and thermal extremes makes this class of materials promising candidates for next-generation advanced structural materials. This study also gives insight into tuning interfaces for controlling twinning as well as material mechanical and thermal stability. Materials fabrication The ARB technique allows for control over individual layer thicknesses ( h ) spanning four to six orders of magnitude. Advantageously, this scalable technology can continuously produce nanomaterial in bulk form, appropriate for industrial applications. The original materials are one polycrystalline sheet of reactor grade Nb (99.97% pure, ATI-Wah Chang) of thickness h =1 mm and two oxide-free high conductivity Cu sheets (99.99% pure, Southern Copper and Supply) of thickness h =0.5 mm, and both of the Cu and Nb sheets are 20-cm long and 6.5-cm wide. After a surface cleaning treatment consisting of a 5-min ultrasonic acetone bath followed by wire brushing to foster bonding, the Cu and Nb sheets were stacked in a sandwich-like structure for the first roll bonding. A 2-high rolling mill (Waterbury-Farrel, Brampton, Ontario, Canada) performed a roll bonding step with an ~60% reduction in layer thickness at room temperature. Then the sample was halved, cleaned and restacked, whereupon the ARB process continued by repeating the steps. The RD was kept unchanged throughout the process. Starting from individual layer thickness of 200 nm, the samples were only subjected to conventional rolling, that is with no cutting and restacking steps, and a usual 10% decrease in total sample thickness per rolling step. Finally, samples with layer thicknesses of 200, 135, 50, 30, 20 and 10 nm were obtained. Neutron diffraction measurements of texture Texture measurements via neutron diffraction were carried out at room temperature on a high pressure preferred orientation [32] time-of-flight diffractometer at the Los Alamos Neutron Science Center at the Los Alamos National Laboratory. The prepared sample was a 1.5-cm 2 coupon of material that was glued to a notched sample holder with the interfaces perpendicular to the incoming neutron beam and the RD of the sample parallel with the notch. Diffraction data were collected from five banks of detector panels set at 2 θ =150°, 120°, 90°, 60° and 40° with each bank creating a full rotation (with regards to neutron beam direction) of detection coverage. To increase the coverage of the pole figures, the sample was rotated to angles of ω =0°, 67.5° and 90°. The MAUD [32] program was used to perform a Rietveld refinement on the 150 neutron diffraction patterns. The Rietveld refinement made use of an E-WIMV method with a 10°-resolution in order to simultaneously fit all the diffraction patterns and determine an orientation distribution function (ODF). The Matlab-based mtex program was then used to rotate the ODF so that the rolling, normal and TDs were properly aligned. In addition, mtex was used to analyze the ODFs and plot the IPFs. TEM characterization TEM samples were prepared by a conventional cross-sectioning method, consisting of low-speed saw cutting, mechanical polishing, dimpling, and ion milling on a Gatan precision ion polishing system operated at 3.5 kV. TEM was performed on a Cs-corrected Titan 80–300 (FEI) operated at 300 kV. All the TEM samples were observed in the TD direction, so that the RD and ND form the viewing plane. Annealing Annealing was performed at a temperature of 500 °C for 1 h in vacuum (4E−06 Torr). The sample was cooled under vacuum. Hardness test Material hardness before and after annealing was measured using nano-indentation on a Nanoindenter XP (Agilent). Indents were performed to a depth of 2000, nm with a target strain rate of 0.05 s −1 . Hardness measurements were made continuously in the continuous stiffness measurement mode. Average hardness values were calculated from 25 separate indents including hardness data from 1,500 to 2,000 nm depths. In all cases, hardness values plateaued in the 1,500–2,000 nm range indicating that a steady-state hardness value had been found. Assumptions that could affect the accuracy of the hardness measurements include an accurate tip area function and an accurate displacement at which the indenter head makes contact with the sample. A silica standard was utilized before and after indentation occurred on each sample in order to ensure an accurate tip area function for the Berkovich tip used. In addition, the onset of loading (an indicator of displacement into sample) was checked for each indent. Geometric phase analysis The GPA method is based on the theory reported by Hytch et al . [42] . A g 1-1-1Cu and a g 1-10Nb were used to produce the strain map. In general, lattice parameters of Cu and Nb in the regions far enough from the interface are consistent with that of bulk materials. Using the average lattice parameter of Cu and Nb as a reference, the tension strain in Nb is ~+5%, and the compression strain in Cu is approximately ~−5%. The strain values in the scale bar are extrapolated according the strain intensity in the map relative to that of the bulk Cu and Nb. The strain map shows that the strains near the interface are nearly zero in between the misfit dislocations, indicating a degree of coherency in those areas and, in principle, the interface misfit dislocations account for the misfit between Cu and Nb. MD simulation The interface formation energy of each interface in Fig. 3e was calculated using molecular dynamics (MD) simulation following the procedures in our previous work [37] , [50] . The energies presented correspond to the relaxed equilibrium atomic structure of the interface predicted by MD. When the Cu and Nb crystals with a given orientation relationship and interface plane are joined, they are allowed to rigidly translate in all x , y and z directions to achieve a structure of minimum interface formation energy. The interface structure is then dynamically relaxed via simulated annealing by lowering the temperature from 300 to 100 K during 60 ps. Once the temperature is lower than 100 K, a subsequent conjugate gradient method is applied. The interface formation energy γ is defined as where the interface region is labelled as I , E i is the potential energy of an atom i , α ( i ) is the species of atom i , is the cohesive energy of species α and A is the interfacial area. Specific details for each interface in Fig. 3e are provided in the Supplementary Method . How to cite this article: Zheng, S. et al . High-strength and thermally stable bulk nanolayered composites due to twin-induced interfaces. Nat. Commun. 4:1696 doi: 10.1038/ncomms2651 (2013).